Implementation of stable and complex biological systems through recombinase-assisted genome engineering Evaluating the performance of engineered biological systems with high accuracy and precision is nearly impossible with the use of plasmids due to phenotypic noise generated by genetic instability and natural population dynamics. Minimizing this uncertainty therefore requires a paradigm shift towards engineering at the genomic level. Here, we introduce an advanced design principle for the stable instalment and implementation of complex biological systems through recombinase-assisted genome engineering (RAGE). We apply this concept to the development of a robust strain of Escherichia coli capable of producing ethanol directly from brown macroalgae. RAGE significantly expedites the optimal implementation of a 34 kb heterologous pathway for alginate metabolism based on genetic background, integration locus, copy number and compatibility with two other pathway modules (alginate degradation and ethanol production). The resulting strain achieves a ~40% higher titre than its plasmid-based counterpart and enables substantial improvements in titre (~330%) and productivity (~1,200%) after 50 generations. In recent years, we have seen rising interest in harnessing the power of microbes for a variety of applications, including engineering pathways for renewable fuel and chemical production [1] , [2] , [3] , [4] , understanding fundamental biological functions (biosensors, gene circuits and rewiring molecular scaffolds) [5] , [6] , and studying multigene and genome-wide molecular genetics [7] , [8] . In synthetic biology, most ventures proceed through four phases of strain engineering—design, construction, implementation (booting) and troubleshooting (debugging) [7] . The design of increasingly more complex biological systems has been greatly enhanced by the wide array of tools now available for controlling heterologous protein and pathway expression at both the transcriptional (promoter and messenger RNA) and translational (RBS) levels [9] , [10] , [11] . Similarly, the construction of large and complex designs has become an almost routine process through the use of cheap, automated and sophisticated techniques for both de novo DNA synthesis [12] , [13] and genetic parts assembly [14] , [15] , [16] , [17] . Despite this unprecedented level of genetic control, however, most engineered systems still do not perform as expected when first implemented in a microbial host. Thus, an additional phase for troubleshooting and debugging is often required to generate genetic diversity and select for improvements in the desired biological function. Due to the cumbersome nature of the implementation and debugging process, most synthetic biology endeavours still rely on plasmid-borne protein expression. However, while the ease of manipulating and transferring extrachromosomal DNA makes plasmids an attractive tool for cursory proof-of-concept studies, their use introduces severe inaccuracies when carefully evaluating the performance of engineered biological systems. Indeed, the combined metabolic burden of both plasmid propagation/maintenance [18] , [19] and pathway overexpression often results in segregational or genetic population events promoting plasmid loss or allele inactivation [20] . In addition, several studies have shown that cell-to-cell variability in copy number can be significant under different cellular growth states and conditions [21] , [22] , a phenomenon that can lead to erratic strain performance. Clearly, the use of stable, integrated components is needed to be able to accurately and precisely assess phenotypic functionality and performance. Unfortunately, the development of efficient, flexible and specific tools for genome engineering, particularly for manipulating and integrating large, complex schemes, is still in its infancy and has hampered progress in the field of synthetic biology. Homologous recombination of single or double-stranded DNA fragments (also called ‘recombineering’) works well for smaller genetic fragments but is cumbersome for larger ones due to both natural limitations in the construction or PCR amplification of long linear fragments and the considerably lower efficiency of integration for inserts greater than just a few kilobases [23] , [24] , [25] . Using this technique, the genomic incorporation of a large multigene pathway would require several sequential rounds of integration and would be a time-consuming and laborious process. Phage integration methods based on recombination between attP – attB sites have higher integration efficiencies and can easily accommodate large plasmid-based fragments [26] , [27] . However, they provide little flexibility over location, as integration is typically limited to existing att sites within the bacterial chromosome. Phage integration also does not allow one to control the specific fragments that are incorporated into the genome; the entire donor plasmid is assimilated, including extraneous genetic components such as the origin of replication. More recently, I-SceI recognition sites have been used to generate double strand DNA breaks in order to mediate site-specific integrations within the chromosome [28] . However, this technique was only demonstrated for a maximum fragment size of 7 kb and is additionally limited to only a single round of incorporation within the same host cell. Here, we describe an advanced design paradigm for the stable and optimal implementation of complex biological systems through recombinase-assisted genome engineering (RAGE). Although RAGE offers broad utility for many areas of biology (that is, it is heavily used in genetics studies of higher organisms [29] , [30] ), the efficiency, flexibility, specificity and speed of recombination make it a disruptive technology for synthetic biology. A detailed schematic of its application to strain implementation is described in Fig. 1 . First, the biological system of interest is constructed on a single copy plasmid or bacterial artificial chromosome (BAC) using various cloning or assembly techniques [12] , [13] , [14] , [15] , [16] , [17] and then transformed into different hosts for proof-of-concept studies aimed at identifying genetic backgrounds that yield the desired phenotype. (Single copy plasmids or BACs are recommended at this step, as they can maintain large DNA fragments at copy numbers that are representative of genome-based expression.) Most strain engineering endeavours do not proceed beyond this step due to technical limitations inherent to genome engineering [31] ; however, the use of RAGE not only allows for the stable instalment of large, complex biological systems, but, more importantly, also enables a full exploration of various parameters, including genetic background, integration locus/location and copy number. Due to the number of strain variants that may need to be generated, efficiency and simplicity are key assets of RAGE, particularly when the performance of the targeted biological system is dependent on other enzymes or genetic modules requiring parallel optimization [32] , [33] . As an added benefit, a stably integrated strain is also much more amenable to additional iterations of strain engineering, including directed or adaptive evolutionary processes aimed at improving phenotype [4] , [8] , [20] . We demonstrate the practical application of this method through the installation and optimization of a 34 kb heterologous gene cluster enabling alginate degradation and utilization in E. coli . The resulting strains are capable of producing ethanol from macroalgae-derived sugars for up to 50 generations at significantly higher titres and productivities over their plasmid-based counterparts. 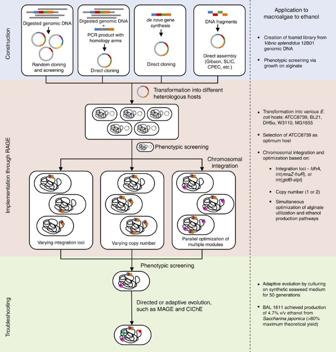Figure 1:Advanced design principle based on the optimal implementation of complex biological systems through RAGE. Top: Construction of biological systems (assembly of genetic parts): A plasmid containing genes responsible for a designed biological function is constructed from either genomic DNA,de novosynthesized DNA and/or DNA fragments through random cloning (library construction), direct cloning or DNA assembly methods12,13,14,15,16,17. Middle: Implementation through RAGE (host strain selection and genome engineering): The expression vector is transformed into different heterologous hosts to identify the specific genetic backgrounds yielding the most desirable cellular phenotypes. Using RAGE, complex biological systems can be integrated into the bacterial genome to explore the effects of integration loci and copy number on phenotype. The efficiency of RAGE also allows for the parallel optimization of multiple genetic modules. Bottom: Troubleshooting desired biological functions (directed and adaptive evolution): The resulting strain can be subjected to additional optimization, including directed or adaptive evolutionary techniques aimed at increasing integrated copy numbers (chemically inducible chemical evolution, CIChE20) or fine-tuning biological function at the genomic level (multiplex automated genome engineering, MAGE8). Classical adaptive evolution approaches can also be applied to improve the desired phenotype. The panel on the right demonstrates the application of RAGE towards engineering macroalgae utilization inE. colifor the production of ethanol. Figure 1: Advanced design principle based on the optimal implementation of complex biological systems through RAGE . Top: Construction of biological systems (assembly of genetic parts): A plasmid containing genes responsible for a designed biological function is constructed from either genomic DNA, de novo synthesized DNA and/or DNA fragments through random cloning (library construction), direct cloning or DNA assembly methods [12] , [13] , [14] , [15] , [16] , [17] . Middle: Implementation through RAGE (host strain selection and genome engineering): The expression vector is transformed into different heterologous hosts to identify the specific genetic backgrounds yielding the most desirable cellular phenotypes. Using RAGE, complex biological systems can be integrated into the bacterial genome to explore the effects of integration loci and copy number on phenotype. The efficiency of RAGE also allows for the parallel optimization of multiple genetic modules. Bottom: Troubleshooting desired biological functions (directed and adaptive evolution): The resulting strain can be subjected to additional optimization, including directed or adaptive evolutionary techniques aimed at increasing integrated copy numbers (chemically inducible chemical evolution, CIChE [20] ) or fine-tuning biological function at the genomic level (multiplex automated genome engineering, MAGE [8] ). Classical adaptive evolution approaches can also be applied to improve the desired phenotype. The panel on the right demonstrates the application of RAGE towards engineering macroalgae utilization in E. coli for the production of ethanol. Full size image Chromosomal integration of large DNA fragments through RAGE In this specific implementation of RAGE, we make use of the Cre recombinase and mutated lox site pairings [29] , [30] , [34] , [35] , [36] to facilitate integration of large genetic fragments into a precise and predetermined location within the bacterial genome ( Fig. 2a ). In the first step of the process, the host or recipient strain is modified by introducing a lox site-flanked antibiotic marker, or ‘targeting cassette,’ at the location of the desired integration. Here, a chloramphenicol resistance gene ( cat ) flanked by loxP and lox5171 sites [34] was integrated using standard λ-RED recombination protocols [23] . In the second step, Cre recombinase expression is induced from the plasmid pJW168 (Lucigen) in order to direct the transfer of a similarly lox -flanked fragment and marker into the genome. This ‘integration cassette’ can be provided on a single-copy plasmid or BAC pre-transformed into the recipient strain (plasmid delivery) or transferred via phage transduction (phage delivery). For the latter option, P1 vir phage lysates are prepared from a donor strain containing the genetic fragment (either on a single or multicopy plasmid or present within the genome) and subsequently used to infect a recipient strain induced for Cre recombinase expression. In the following examples, an FRT-flanked kanamycin resistance gene ( kan ) was included in the cassette to select for proper integration events. Excision of kan through expression of the FLP recombinase [23] allows for the generation of markerless integration strains capable of undergoing additional rounds of genetic modification. 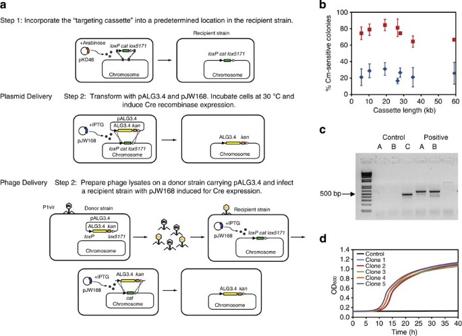Figure 2:Recombinase-assisted genome engineering (RAGE). RAGE is a genome engineering strategy that facilitates stable instalment and implementation of complex biological systems by recombinase-mediated cassette exchange. (a) In the first step, thecatgene flanked by two mutually exclusiveloxsites (‘targeting cassette’) is incorporated into the bacterial genome through arabinose induction of the λ-RED recombination genes (on pKD46). With plasmid delivery, this strain is subsequently transformed with both pJW168 and the donor plasmid carrying thelox-flanked genetic fragment (in this case, pALG3.4), then grown at 30 °C with IPTG to induce Cre recombinase expression. With phage delivery, P1virlysates are prepared from a recipient strain containing pALG3.4 and subsequently used to infect a recipient strain induced for Cre recombinase expression. In both cases, the temperature-sensitive plasmid pJW168 is lost following plating on kanamycin and growth at 37 °C. (b) Relationship between integration efficiency and cassette length. Efficiency is represented as the percent of kanamycin-resistant colonies that also exhibited sensitivity to chloramphenicol by either plasmid delivery (red squares) or phage delivery (blue diamonds). Error bars represent s.d. from at least three replicate platings. (c) Colony PCR verification of integrated strains across the ldhA junction. BAL 1075ldhA::loxP-cat-lox5171was used as a negative control for the PCR reactions. Expected product sizes are as follows—A (left end verification): 588 bp; B (right end verification): 608 bp; C (ldhA::loxP-cat-lox5171cassette): no product expected if correct or 471 bp if integration failed. Because similar results were found for all 10 strains tested, only one representative set is shown. (d) Growth of five integration clones on 2% degraded alginate medium. BAL 1075 was used as a negative control for these growth assays. Clones 1–3 were derived through the plasmid delivery method, and clones 4–5 were obtained through phage delivery. Figure 2: Recombinase-assisted genome engineering (RAGE) . RAGE is a genome engineering strategy that facilitates stable instalment and implementation of complex biological systems by recombinase-mediated cassette exchange. ( a ) In the first step, the cat gene flanked by two mutually exclusive lox sites (‘targeting cassette’) is incorporated into the bacterial genome through arabinose induction of the λ-RED recombination genes (on pKD46). With plasmid delivery, this strain is subsequently transformed with both pJW168 and the donor plasmid carrying the lox -flanked genetic fragment (in this case, pALG3.4), then grown at 30 °C with IPTG to induce Cre recombinase expression. With phage delivery, P1 vir lysates are prepared from a recipient strain containing pALG3.4 and subsequently used to infect a recipient strain induced for Cre recombinase expression. In both cases, the temperature-sensitive plasmid pJW168 is lost following plating on kanamycin and growth at 37 °C. ( b ) Relationship between integration efficiency and cassette length. Efficiency is represented as the percent of kanamycin-resistant colonies that also exhibited sensitivity to chloramphenicol by either plasmid delivery (red squares) or phage delivery (blue diamonds). Error bars represent s.d. from at least three replicate platings. ( c ) Colony PCR verification of integrated strains across the ldhA junction. BAL 1075 ldhA :: loxP - cat - lox5171 was used as a negative control for the PCR reactions. Expected product sizes are as follows—A (left end verification): 588 bp; B (right end verification): 608 bp; C ( ldhA :: loxP - cat-lox5171 cassette): no product expected if correct or 471 bp if integration failed. Because similar results were found for all 10 strains tested, only one representative set is shown. ( d ) Growth of five integration clones on 2% degraded alginate medium. BAL 1075 was used as a negative control for these growth assays. Clones 1–3 were derived through the plasmid delivery method, and clones 4–5 were obtained through phage delivery. Full size image Advantages of RAGE The utility of RAGE was first demonstrated through the incorporation of a 34 kb alginate metabolic pathway (from pALG3.4, a modified version of pALG3 (ref. 37 )) into the ldhA locus of BAL 1075 ( Table 1 ) ( Fig. 2b–d ). Strains that have successfully undergone fragment integration into the targeted locus should exhibit both kanamycin resistance and chloramphenicol sensitivity (conferred by the loss of cat through cassette replacement), thus providing a simple initial screen for recombination accuracy ( Fig. 2b ). Indeed, colony PCR verification of the ldhA junctions revealed correct fragment placement in all 10 chloramphenicol-sensitive strains tested ( Fig. 2c ). Because of the large size of the integration cassette, fragment integrity was tested through growth on alginate-derived medium rather than through resequencing of the entire genetic construct. Although innocuous mutations cannot be detected through this assay, insertions, deletions or point mutations that alter protein function should be reflected as a shift in the growth properties of the strains. As shown in Fig. 2d , however, five individual colonies exhibited similar growth profiles on 2% degraded alginate medium, indicating a low rate of mutation within the genetic fragment. (The likelihood of introducing point mutations remains low, as genetic fragments are incorporated directly from the donor material without the need for PCR amplification.) The five clones tested were obtained by both plasmid and phage delivery of the integration cassette, demonstrating that the use of either methodology leads to 100% cassette integrity and functionality after selecting for kanamycin resistance and chloramphenicol sensitivity. These results suggest that a simple antibiotic screen is sufficient for obtaining a proper integrant. After engineering lox sites flanking the donor region of interest, the entire integration procedure can be implemented and confirmed in under a week. Table 1 Strains used in this study. Full size table Homologous recombination-based techniques for genomic integration are widely used in bacterial engineering but often exhibit very low efficiencies, particularly for cassettes greater than just a few kilobases in length [34] . As such, they often require a cumbersome validation process to select for a correct integrant. To determine the effect of cassette size on the performance of our method, we constructed several alternate versions of pALG3 containing partial or extended alginate pathways ranging from 5.6 kb to 59 kb in length ( Table 2 ). Efficiencies of integration and correct cassette localization were then determined based on the percent of recovered (kanamycin-resistant) colonies exhibiting chloramphenicol sensitivity (although we note that selected colonies from each cassette length were additionally verified by performing colony PCR across the integration junctions). As shown in Fig. 2b , the phage delivery method showed no dependence on length with efficiencies ranging between 20–30% across all fragment sizes. Efficiencies with plasmid delivery were much higher (65–85%) and showed only a slight drop for cassettes greater than 30 kb. Because the 59 kb fragment comprises an extended alginate pathway containing additional copies or orthologs of several alginate degradation enzymes, strains with a correctly integrated cassette should display enhanced growth properties over its 34 kb counterpart. Indeed, strains with the extended pathway displayed both higher growth rates (μ=0.34 per hour versus 0.30 per hour) and maximum cell densities (OD 600 =1.6 versus 1.1) when grown on 2% degraded alginate medium. Thus, this methodology can be utilized for the integration of cassette sizes up to at least 59 kb with both high accuracy and efficiencies. Table 2 Constructed pALG plasmid versions and their corresponding lox -flanked cassette sizes. Full size table Efficient and optimal implementation of biological systems To demonstrate the potential of the advanced design principle, we applied it towards engineering a microbial platform for the conversion of brown macroalgae (brown seaweed) into ethanol ( Fig. 1 ). Brown macroalgae possess several attractive features, which make them ideal next-generation feedstocks for biofuel and chemical production [37] . Unlike sugarcane or corn, seaweed cultivation does not require arable land, fertilizer or fresh water resources, thus minimizing its impact on both the environment and existing food supplies. The absence of lignin in seaweed also eliminates the requirement for expensive pretreatment operations to promote sugar release. Although E. coli readily utilizes two of the three main sugars in seaweed—mannitol and glucan (glucose polymers in the form of laminarin or cellulose)—no industrial strain to-date has the capability of metabolizing the third sugar component, alginate. We have previously shown that efficient utilization of alginate requires a 34 kb heterologous gene cluster from Vibrio splendidus 12B01 present on the single-copy plasmid pALG3 (originally constructed by using recombineering techniques on the fosmid pALG1, which was isolated from a genomic library of V. splendidus 12B01) [37] . To determine the optimal strain for this pathway, we first transformed pALG3 into five E. coli variants –ATCC 8739, BL21, DH5α, K-12 (MG1655) and W3110. Growth on 2% degraded alginate was then used as a crude readout for pathway expression and functionality. Although the presence of pALG3 was able to impart growth on alginate for all five genotypes tested, ATCC 8739 exhibited a much faster growth rate and was therefore selected for subsequent integration studies ( Fig. 3a ). 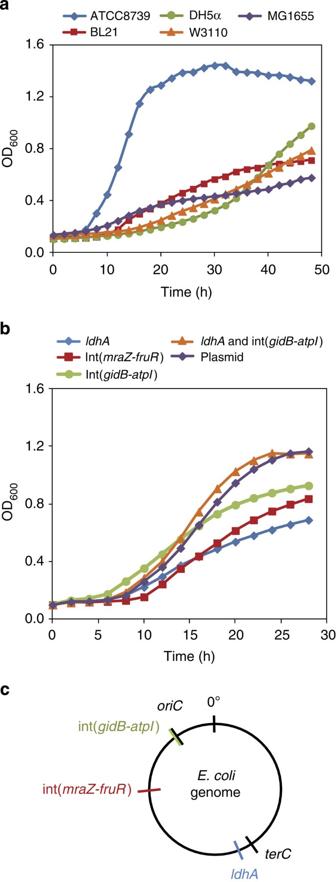Figure 3: Growth of strains on 2% degraded alginate. (a) pALG3 in five differentE. colistrain backgrounds (b) Integration of ALG3.4 into different loci withinE. coliATCC8739’s genome. Data points represent averages from at least three biological replicates. All standard deviations were less than 5% of the average, and error bars have been omitted for visual clarity. (c) Positioning of three integration loci relative to theoriCand the terminus of replication (terC) of theE. coligenome. Figure 3: Growth of strains on 2% degraded alginate. ( a ) pALG3 in five different E. coli strain backgrounds ( b ) Integration of ALG3.4 into different loci within E. coli ATCC8739’s genome. Data points represent averages from at least three biological replicates. All standard deviations were less than 5% of the average, and error bars have been omitted for visual clarity. ( c ) Positioning of three integration loci relative to the oriC and the terminus of replication ( terC ) of the E. coli genome. Full size image Because chromosomal positioning has been shown to have a role in gene expression [38] , we explored loci-dependent transcriptional variation by integrating our pathway into three different locations within the ATCC 8739-derived strain, BAL 1075 ( Table 1 ). The following positions were selected based on their distance to the chromosomal origin of replication ( oriC ): (1) the intergenic region of gidB and atpI (0.1% away from oriC ), (2) the intergenic region of mraZ and fruR (33.3% away from oriC ) and (3) ldhA (99.5% away from the oriC ). In this context, percent distance represents the fraction of the genome that is closer to the oriC . As chromosomal replication begins at oriC , genes that are located near this reference point are duplicated first and possess a higher ‘effective copy number’ within the cell [38] . As seen in Fig. 3b , we found a clear negative correlation between growth and distance from oriC , confirming that the best expression can be obtained at locations closer to the origin of replication. Interestingly, the growth of even the best single-copy integration (in the intergenic region of gidB and atpI ) still lagged in comparison to a strain carrying the single-copy plasmid, pALG3. These differences were largely eliminated through the introduction of a second copy of the alginate pathway into the ldhA locus via phage transduction. Parallel optimization of a multi-module microbial system Although two integrated copies of the alginate metabolic pathway are clearly needed for robust growth on degraded alginate, phenotypes that divert cellular resources from biomass generation into alternate products may possess different expression level optima. As an example, we postulated that efficient production of ethanol from alginate may require balancing of the two pathway modules for alginate consumption and the conversion of pyruvate to ethanol. To determine the most effective coupling of alginate utilization and ethanol production, we constructed and tested the full matrix of single and double integrations for each independent module ( Table 3 ). The alginate metabolic pathway from pALG3 was incorporated into the intergenic regions of mraZ and fruR (single copy) and gidB and atpI (double copy). To engineer robust ethanol production, the homoethanol pathway encoded by the Zymomonas pyruvate decarboxylase (Pdc) and alcohol dehydrogenase B (AdhB) genes was integrated as a single copy ( frd locus, controlled by the strong constitutive promoter P G25 from phage T5 in BAL 1303 ( Table 1 )) or as double copies ( frd / pta / focA-pflB loci in BAL 1075 controlled by their native promoters). We also expressed a secretable alginate lyase system on the single-copy plasmid N455+tSM0524 Aly to catalyse the extracellular depolymerization of alginate [37] . Table 3 Strains generated for the comparison of plasmid- and chromosomal-based expression for three independent genetic modules. Full size table To evaluate their performance, strains were grown microaerobically in synthetic seaweed media containing 50 g l −1 total sugars (alginate, mannitol and glucose at a ratio of 5:8:1) and assayed for ethanol production (maximum theoretical titre of ethanol is 25 g l −1 ). In all cases, we observed lower ethanol titres ( Fig. 4a ) and productivities ( Fig. 4b ) in strains harbouring a plasmid-based alginate pathway relative to their integrated counterparts ( P <0.001 by Student’s t -test), indicating that plasmid instability is an issue, even at these shorter time scales. (The only exception is BAL 1452, which seems to be impaired by the overexpression of enzymes from double chromosomal copies of both the ethanol and alginate pathways.) Although both BAL 1075 and BAL 1303 possess the ability to produce ethanol from glucose with nearly theoretical maximum yield, ethanol production is significantly reduced in BAL 1075 with an integrated alginate pathway, thus highlighting the importance of optimizing relative expression levels through empirical testing. The best overall performance was obtained from two strains containing a single integrated ethanol pathway and either one or two copies of the alginate pathway (BAL 1450 and BAL 1493, respectively), yielding titres of 21–22 g l −1 ethanol (83–87% of the maximum theoretical yield) and productivities of 0.35 g l/h. Integration of the secretable alginate lyase system from N455+tSM0524 Aly into BAL 1450 yielded BAL 1611, a fully integrated strain possessing an ~40% improvement in ethanol production over its plasmid-based counterpart BAL 1373 ( Fig. 4 ). 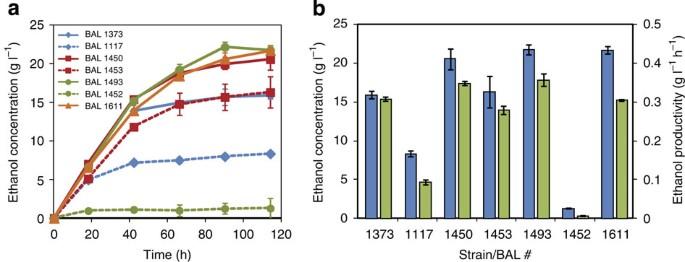Figure 4: Effect of plasmid- and chromosomal-based expression on ethanol production. Strain numbers correspond toTable 1. (a) Ethanol production profiles—Matching colours represent strains with identical alginate lyase and alginate pathway configurations with either a single integrated copy (solid line) or two integrated copies (dashed line) of the ethanol pathway. (b) Final ethanol titres (114 h, blue) and productivities (18–42 h, green). Error bars represent standard deviations from at least three biological replicates. Figure 4: Effect of plasmid- and chromosomal-based expression on ethanol production. Strain numbers correspond to Table 1 . ( a ) Ethanol production profiles—Matching colours represent strains with identical alginate lyase and alginate pathway configurations with either a single integrated copy (solid line) or two integrated copies (dashed line) of the ethanol pathway. ( b ) Final ethanol titres (114 h, blue) and productivities (18–42 h, green). Error bars represent standard deviations from at least three biological replicates. Full size image Stable maintenance of phenotype over 50 generations From an industrial context, strain implementation through RAGE is especially advantageous, as it allows for the extended maintenance of phenotypes, even in the absence of external selection pressures such as antibiotics. To assess the genetic and phenotypic stability of our engineered strains, BAL 1373, BAL 1450 and BAL 1611 were grown in synthetic seaweed media over 50 generations through 11 successive rounds of serial subculturing. Strains that retain their properties through 50 doublings are expected to remain stable from a seed inoculum all the way up to an industrial scale process (~150,000 l). Although plasmid-based expression of the alginate pathway in BAL 1373 was already previously shown to be unfavourable ( Fig. 4 ), extended culturing of this strain in synthetic seaweed media led to an additional twofold drop in final ethanol titre ( Fig. 5a ). In stark contrast, integration of the alginate pathway in both BAL 1450 and BAL 1611 led to stable phenotypes over 50 generations, with strains achieving even slightly higher titres and productivities than the original, unsubcultured variants ( P <0.01 by Student’s t -test) ( Fig. 5b,c ). The performance of BAL 1611 beats its plasmid counterpart BAL 1373 by a significant margin (~330% in titre and ~1,200% in productivity) despite the presence of strong selection pressures (antibiotic supplementation and carbon utilization for growth) to encourage plasmid maintenance. 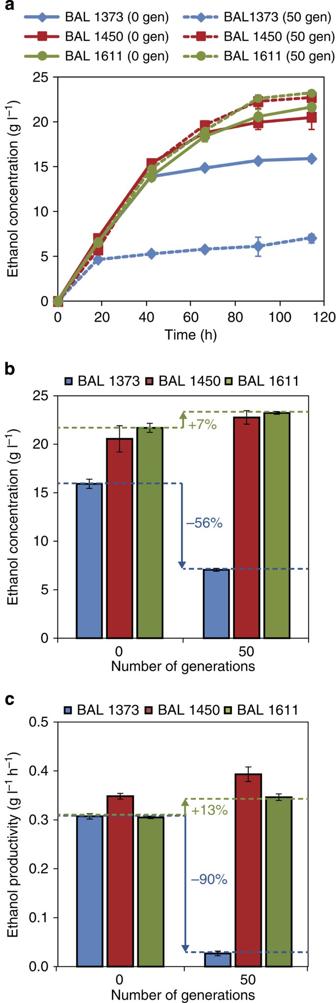Figure 5: Performance of select strains after 0 or 50 generations of culturing. Strain numbers correspond toTable 1. (a) Ethanol production profiles—Matching colours represent identical strains tested after 0 generations (solid line) or 50 generations (dashed line) of culturing. (b) Final ethanol titres (114 h) and (c) ethanol productivities (18–42 h). Error bars represent standard deviations from at least three biological replicates. Figure 5: Performance of select strains after 0 or 50 generations of culturing. Strain numbers correspond to Table 1 . ( a ) Ethanol production profiles—Matching colours represent identical strains tested after 0 generations (solid line) or 50 generations (dashed line) of culturing. ( b ) Final ethanol titres (114 h) and ( c ) ethanol productivities (18–42 h). Error bars represent standard deviations from at least three biological replicates. Full size image Genetic instability and subsequent loss of function can be severe in engineered strains even with the use of single copy, low-metabolic burden expression vectors and multiple routes for selection and plasmid retention. As such, evaluating the performance of engineered biological systems with high accuracy and precision is nearly impossible with the use of plasmid systems. As demonstrated here, RAGE encompasses several important features that make it an enabling technology for many applications within synthetic biology, including the construction and optimization of genetically stable strains. First, the use of a site-specific recombinase such as the Cre enzyme allows for a high efficiency of integration, even for large genetic fragments. Although the maximum size tested in this study was 59 kb, we expect this methodology to have the capacity to incorporate even larger pieces with minimal impact on efficiency. Phage delivery can mediate the insertion of pieces up to 90 kb in size, an upper bound imposed by the amount of DNA packaged into the head of a bacteriophage particle [39] . Plasmid delivery has even less stringent limitations as it only requires stable maintenance of the genetic fragment on a plasmid or BAC, the latter of which has been routinely used for genetic fragments as large as 300 kb in size [40] . Second, RAGE is versatile and flexible with respect to both integration locus (determined through placement of the targeting cassette) and mode of fragment delivery (phage or plasmid). Although our efficiency studies revealed a two- to fourfold higher rate of integration via (single copy) plasmid delivery ( Fig. 2b ), phage delivery allows for the insertion of fragments that reside within a chromosome or on a multicopy plasmid, thus expanding the array of acceptable donor material. A third important feature of this method is its ability to maintain cassette integrity during chromosomal incorporation, even for large constructs. Due to the size of our alginate utilization pathway, direct sequencing of the genetic cluster would have been both expensive and impractical. We therefore used growth rates on 2% degraded alginate as surrogate readout to verify cassette integrity and found very close agreement among several colonies that were tested ( Fig. 2d ). Indeed, the likelihood of introducing point mutations remains low, as genetic fragments are incorporated directly from the donor material without the need for PCR amplification. Taken altogether, the efficiency, specificity and speed of RAGE pave the way for an advanced design paradigm for the stable and optimal implementation of complex biological systems, facilitating explorations based on several genetic parameters, including strain background, integration loci and copy number. The potential of this method is most palpable when working with long heterologous pathways, particularly in situations when cellular phenotype is dependent on two or more modules requiring parallel optimization. Although RAGE was only applied towards integration of a single module in this example, it is a straightforward exercise to pursue the integration of multiple modules into a variety of backgrounds through the use of alternate mutually exclusive lox site pairings [34] , [35] , [36] . Finally, coupling this technique with adaptive evolution or direct genome editing [4] , [8] , [20] can further optimize the performance of the designed biological functions of interest. Indeed, the recovery of better ethanol producers after 50 generations of culturing clearly demonstrates the potential of generating additional improvements in phenotype through adaptive evolution and screening. Given such advantages, we expect the application of RAGE and this implementation paradigm to significantly accelerate the exploration of many more avenues within synthetic biology. As we have previously reported, the fully integrated strain BAL 1611 generated by this study has proven to be well-optimized and is capable of producing 4.7% v/v ethanol (over 80% of the maximum theoretical yield) directly from brown macroalgae with a yield of 0.281 g-ethanol/g-dry seaweed [37] . This efficient utilization of macroalgae sugars coupled with its enhanced genetic stability make this strain a suitable microbial platform for the industrial-scale production of renewable fuels and chemicals from seaweed. Cultivation conditions All strain/plasmid manipulations were conducted on Luria-Bertani (LB) medium. When appropriate, antibiotics were added at the following concentrations: 25 μg ml −1 chloramphenicol for maintenance of cat -containing plasmids or strains, 12.5 μg ml −1 kanamycin for maintenance of kan -containing plasmids or strains and 100 μg ml −1 ampicillin for maintenance of pKD46, pCP20 and pJW168. Primers used in this study are listed in Supplementary Table S1 . Modification of pALG plasmids for Cre- lox recombination Two lox sites— loxP and lox5171 —were introduced into pALG3 (ref. 37 ) through four rounds of sequential modifications with λ-RED recombination [23] . pALG3.1 was constructed by amplifying cat from pCm-R6Kγ [41] with primers CS009 Cm/Km hom sense and CS010 Cm anti-hom and transforming the resulting cassette into DH5α pALG3 pKD46 electrocompetent cells. This initial step was necessary to change the antibiotic resistance of pALG3 from kanamycin to chloramphenicol ( kan to cat ) in order to facilitate downstream integration steps. To insert a loxP site into pALG3.1 (to form pALG3.2), the loxP :: kan FRT cassette was amplified from pKD13 with primers CS037 hom-pKD13 sense and CS038 hom-loxP-pKD13 anti, followed by a second round of amplification with CS039 pKD13 sense 2 and CS040 lox-pKD13 anti 2. Excision of FRT-flanked kan was mediated by transformation with the FLP recombinase-expressing plasmid pCP20 (ref. 23 ) to form pALG3.3. In the final step of modification, a lox5171 site was introduced into pALG3.3 by amplifying a lox5171 :: kan FRT cassette from pKD13 with primers CS011 lox5171-pKD13 anti and CS013 hom1-pKD13 sense, followed by a second round of amplification with CS012 lox5171-pKD13 anti 2 and CS013 hom1-pKD13 sense. The cassette was subsequently transformed into DH5α pALG3.3 pKD46 to form pALG3.4, a plasmid containing a 35 kb fragment flanked by loxP , lox5171 and kan FRT . Plasmids pALG3.5–8 were additionally constructed to provide integration cassettes of varying lengths, ranging from 5.6 kb to 26.5 kb. lox5171 :: kan FRT cassettes for construction were amplified with CS011 lox5171-pKD13 and CS014-17 hom2-5 pKD13 sense, followed by a second round of amplification with CS012 lox5171-pKD13 anti 2 and the same set of second primers. Cassettes were subsequently transformed into DH5α pALG3.3 pKD46. Two lox sites— loxP and lox5171 —were introduced into pALG4 to yield pALG4.4 through a similar method as described above. CS037 hom-pKD13 sense-CS115 hom-loxP-pKD13 anti and CS039 pKD13 sense 2-CS116 lox-pKD13 anti 2 primer pairings were used to amplify the loxP :: kan FRT cassette from pKD13 for the construction of pALG4.2. Excision of FRT-flanked kan was mediated by transformation with pCP20 to form pALG4.3, and the lox5171 :: kan FRT cassette was amplified from pKD13 with primer pairs CS011 lox5171-pKD13 anti -CS120 hom-pKD13 sense and CS012 lox5171-pKD13 anti 2 -CS120 hom-pKD13 sense to form pALG4.4. Two lox sites— loxP and lox5171 —were introduced into pALG7 to yield pALG7.4. Construction of pALG7.8.2 and pALG7.8.3 proceeded through the same steps as for pALG3.2 and pALG3.3. The lox5171 :: kan FRT cassette was amplified from pKD13 with primer pairs CS011 lox5171-pKD13 anti-CS113 hom-pKD13 sense and CS012 lox5171-pKD13 anti 2-CS113 hom-pKD13 sense to form pALG7.4. Correct integration events were verified after each step by colony PCR and sequencing. Construction of BAL1075 To achieve stable ethanol production, pdc and adhB derived from Zymomonas mobilis ( Zm _ pdc and Zm _ adhB ) and pdc derived from Zymomonas palmae ( Zp _ pdc ) were integrated into the E. coli host ATCC8739 Δ ldhA [37] . Briefly, DNA fragments for Zm _ adhB and the FRT-flanked kanamycin cassette from pKD13 ( kan FRT )were first amplified from Z. mobilis genomic DNA and pKD13 using forward primers adhB-pKD13-F and pKD13-F and reverse primers adhB-R and adhB-pKD13R, respectively. Amplified fragments were gel purified and adjoined by PCR using the primer set pKD13-F and adhB-R, then treated with T4 DNA polynucleotide kinase and ligated with T4 DNA ligase to form pKD13- adhB . The Zm _ adhB - kan FRT cassette was amplified from pKD13- adhB using forward primer frd-adhB-F and reverse primer frd adhB-R and integrated into the frd gene locus of E. coli ATCC8739 Δ ldhA via λ-RED recombination [23] to form ATCC8739 Δ ldhA Δ frd :: Zm _ adhB . A similar procedure was used to create pKD13- pdc using forward primers pdc-F and pdc-pKD13-F and reverse primers pdc-pKD13-R and pKD13-R to amplify Zm _ pdc and kan FRT from Z. mobilis genomic DNA and pKD13, respectively. The Zm _ pdc - kan FRT cassette was then amplified from pKD13- pdc using forward primer pta-pdc-F and reverse primer pta-pdc-R and integrated into the pta gene locus of E. coli strain ATCC8739 Δ ldhA Δ frd :: Zm _ adhB via λ-RED recombination to form ATCC8739 Δ ldhA Δ frd :: Zm _ adhB Δ pta :: Zm _ pdc . pKD13-pflPr- Zp_pdc-adhB - kan FRT -pflTm was created by amplifying DNA fragments for the pfl promoter (pflPr), Zp_pdc , Zm_adhB, kan FRT , the pfl terminator (pflTm) and R6Kγ using forward primers pflPr-F, pflPr-Zp_pdc-F, Zp_pdc-adhB-F, adhB-FRT-Km-FRT-F, FRT-Km-FRT-pflTm-F and pflTm-R6Kγ-F and reverse primers Zp_pdc-adhB-R, adhB-FRT-Km-FRT-R, FRT-Km-FRT-pflTm-R, pflTm-R6Kγ-R and R6Kγ-R, respectively. Genomic DNA from E. coli , Z. palmae , and Z. mobilis and pKD13 were used as templates. The amplified fragments were gel purified and adjoined by PCR using the primer set pflPr-F and pflTm-R, then treated with T4 DNA polynucleotide kinase and ligated with T4 DNA ligase to form pKD13-pflPr- Zp_pdc-adhB - kan FRT -pflTm. Zp_pdc-adhB - kan FRT was amplified from this plasmid using forward primer pflPr-F and the reverse primer pflTm-R and integrated into the focA-pflB gene locus of E. coli ATCC8739 Δ ldhA Δ frd :: Zm _ adhB Δpta:: Zm_pdc via λ-RED recombination to form BAL1075 (ATCC8739 Δ ldhA Δ frd :: Zm _ adhB, Δ pta :: Zm _ pdc, Δ focA-pflB :: Zp_pdc-Zm_adhB ). Excision of kan FRT after all integration events was mediated by transformation with the FLP recombinase-expressing plasmid pCP20 (ref. 23 ). Genomic insertion of lox targeting cassette Lox sites were integrated into the ldhA locus of BAL 1075 ( Table 1 ) using λ-RED recombination [23] and a chloramphenicol marker ( cat ). Briefly, cat was amplified from pCm-R6Kγ [41] with primers CS001 lox5171-Cm sense, CS002 loxP-Cm anti and Phusion Hot-Start II DNA polymerase (New England BioLabs). Two distinct and mutually exclusive lox sites ( loxP, lox5171 (ref. 29 )) were incorporated into the primer sequences to allow for double-crossover recombination of similarly lox -flanked fragments into the genome. In addition, these primers contained 28–29 bp homology with the ldhA region of E. coli ATCC 8739. The resulting ldhA :: loxP - cat - lox5171 cassette was then re-amplified with primers CS003 lox-Cm sense 2 and CS004 lox-Cm anti 2 to extend its ldhA homology region (for a total of 78 bp) and subsequently utilized for λ-RED recombination [23] . Lox sites were integrated into the intergenic regions of gidB and atpI and mraZ and fruR through a similar method as above. The int( gidB - atpI ):: loxP-cat-lox5171 integration cassette was amplified with CS095 lox5171-gidB-atpI sense and CS096 loxP-gidB-atpI anti, followed by a second round of amplification with CS097 lox-gidB-atpI sense 2 and CS098 lox-gidB-atpI anti 2. The int( mraZ - fruR ):: loxP - cat - lox5171 cassette was amplified with CS105 lox5171-mraZ-fruR sense and CS106 loxP-mraZ-fruR anti, followed by a second round of amplification with CS107 lox-mraZ-fruR sense 2 and CS108 lox-mraZ-fruR sense 2. Colony selection was performed on LB-agar plates with 25 μg ml −1 chloramphenicol, and correct integration events were verified by colony PCR and sequencing. Cre- lox -mediated integration via plasmid delivery To create BAL 1075 ldhA :: loxP -ALG3.4- lox5171 , BAL 1075 ldhA :: loxP - cat - lox5171 was transformed with pALG3.4 and pJW168 (Lucigen), a plasmid containing a temperature-sensitive replicon and an inducible Cre recombinase. After overnight growth in LB medium at 30 °C, 25 μl was used to inoculate 2.5 ml fresh LB with 1 mM Isopropyl-β- D -thiogalactopyranoside (IPTG) and 12.5 μg ml −1 kanamycin. Cultures were grown for 3–6 h at 30 °C, then streaked out on LB-agar plates with kanamycin to isolate single colonies. After overnight growth at 37 °C, individual colonies were streaked out on LB-kanamycin and LB-chloramphenicol to identify chloramphenicol-sensitive colonies. These colonies were additionally verified for proper end integration by colony PCR using primer pairs CS005 ldhA verif sense-CS063 left verif anti and CS008 ldhA verif anti-CS064 right verif sense. Correct colonies were also streaked out on LB-ampicillin plates to verify loss of pJW168. A similar procedure was used to create strains BAL 1075 int( gidB - atpI ):: loxP -ALG3.4- lox5171 , BAL 1075 int( mraZ - fruR ):: loxP -ALG3.4- lox5171 (BAL 1453), and BAL 1303 int( mraZ - fruR ):: loxP -ALG3.4- lox5171 (BAL 1450). Primers used for colony PCR are as follows: int( gidB-atpI )—CS063 left verif anti-CS099 gidB-atpI verif sense and CS064 right verif sense-CS100 gidB-atpI verif anti; int( mraZ - fruR )—CS064 right verif sense -CS109 mraZ-fruR verif sense and CS063 left verif anti -CS110 mraZ-fruR verif anti. Excision of FRT-flanked kan was mediated by transformation with the FLP recombinase-expressing plasmid pCP20. To test the effect of cassette length on integration efficiency, the same procedure was repeated for pALG3.5–8. Efficiency was defined as the percent of colonies that were found to be chloramphenicol sensitive (out of a total of about 30 colonies). In addition, two random chloramphenicol-sensitive colonies from each culture were chosen for colony PCR verification. Triplicate cultures and recombination experiments were performed for each plasmid version. Cre- lox -mediated integration via phage delivery BAL 1075 was transformed with pALG3.4 and used for the preparation of lysates from the P1 vir bacteriophage [39] , [42] . This lysate was subsequently used to infect an overnight culture of BAL 1075 ldhA :: loxP - cat - lox5171 pJW168 grown at 30 °C in LB medium with ampicillin and 1 mM IPTG. Following a 1-h infection, cells were plated on LB-agar plates with kanamycin to isolate single colonies. After overnight growth at 37 °C, individual colonies were streaked out on LB-kanamycin and LB-chloramphenicol to identify chloramphenicol-sensitive colonies. These colonies were additionally verified for proper end integration by colony PCR using the primer pairs listed above. Correct colonies were also streaked out on LB-ampicillin plates to verify loss of pJW168. Excision of FRT-flanked kan was mediated by transformation with the FLP recombinase-expressing plasmid pCP20. To test the effect of cassette length on integration efficiency, the same procedure was repeated for pALG3.5–8. Efficiency was defined as the percent of colonies that were found to be chloramphenicol sensitive (out of a total of about 30 colonies). In addition, two random chloramphenicol-sensitive colonies from each culture were chosen for colony PCR verification. Triplicate lysate preparation and infection experiments were performed for each plasmid version. Increasing gene copy number through P1 vir phage transduction Transfer of a second integrated copy of ALG3.4 (into BAL 1450 to generate BAL 1493 or into BAL 1453 to generate BAL 1452) was mediated by P1 vir phage transduction [39] , [42] . Proper integration was verified by colony PCR as described above. Excision of FRT-flanked kan was mediated by transformation with the FLP recombinase-expressing plasmid pCP20. Alginate growth assays Strains used for alginate growth assays were first grown overnight in LB medium at 30 °C. Hundred-microliters of cell culture was then washed and resuspended in an equal volume of 2% degraded alginate medium (M9 minimal medium with 2% alginate pre-degraded with 10 μg ml −1 alginate lyase (Sigma) overnight at 30 °C), and 4 μl was used as an inoculum for 196 μl 2% degraded alginate medium. Alginate growth assays were performed at 30 °C, and cell density (OD 600 ) was monitored with a BioTek Synergy HT Multidetection microplate reader. All liquid cultivations were conducted with at least three biological replicates. Ethanol fermentations Ethanol fermentations were conducted in stirred bottles containing 100 ml M9 minimal media with 50 g l −1 sugars (alginate, mannitol and glucose at a ratio of 5:8:1) and 5 g l −1 LB. Cultures were inoculated to a starting cell density (OD 600 ) of ~0.6 and kept at 25 °C. Ethanol concentrations were quantified by high performance liquid chromatography (Shimadzu, Columbia, MD) equipped with an organic acid column (Phenomenex, Torrance, CA). Chromatography was operated at 60 °C using 5 mM H 2 SO 4 as a mobile phase at a flow rate of 1 ml min −1 (5 μl injection volume, 15 min isocratic method). Ethanol peaks were detected using a refractive index detector and compared with chemical standards. How to cite this article: Santos, C.N.S. et al . Implementation of stable and complex biological systems through recombinase-assisted genome engineering. Nat. Commun. 4:2503 doi: 10.1038/ncomms3503 (2013).